Ciliary dysfunction impairs beta-cell insulin secretion and promotes development of type 2 diabetes in rodents Type 2 diabetes mellitus is affecting more than 382 million people worldwide. Although much progress has been made, a comprehensive understanding of the underlying disease mechanism is still lacking. Here we report a role for the β-cell primary cilium in type 2 diabetes susceptibility. We find impaired glucose handling in young Bbs4 −/− mice before the onset of obesity. Basal body/ciliary perturbation in murine pancreatic islets leads to impaired first phase insulin release ex and in vivo . Insulin receptor is recruited to the cilium of stimulated β-cells and ciliary/basal body integrity is required for activation of downstream targets of insulin signalling. We also observe a reduction in the number of ciliated β-cells along with misregulated ciliary/basal body gene expression in pancreatic islets in a diabetic rat model. We suggest that ciliary function is implicated in insulin secretion and insulin signalling in the β-cell and that ciliary dysfunction could contribute to type 2 diabetes susceptibility. The number of people suffering from type 2 diabetes mellitus (T2DM) worldwide is expected to exceed 590 million within one generation (by 2035) [1] . T2DM is a chronic disease with devastating complications and the fifth leading cause of death worldwide [2] . Over the past decade, biomedical research has experienced a renewed interest in the primary cilium and its role as a sensory organelle [3] . Implications of ciliary dysfunction in a subset of human diseases, the ciliopathies, have spurred further investigations of the ciliary role in development and disease [4] . Common clinical features in ciliopathies include retinal dystrophy and renal cysts. Some syndromic ciliopathies that present with severe truncal obesity, such as Bardet–Biedl Syndrome (BBS, Online Mendelian Inheritance in Man accession code 209900) and Alström Syndrome (ALMS, Online Mendelian Inheritance in Man accession code 203800), also have a high co-morbidity with T2DM [5] , [6] . The ciliary axoneme and its proximity to the microtubule-organizing centre seems to provide spatio-temporal organization of several biological signalling cascades and thus represents a point of convergence of these pathways [3] , [7] . In Caenorhabditis elegans , ciliary proteins affect life span and dauer formation and therefore implicate cilia in the insulin/insulin-like growth factor 1 (IGF1)-signalling cascades [8] , [9] . In both mice and humans, primary cilia are found in pancreatic islets on α-, β- and δ-cells and in pancreatic ducts, but they are absent from the exocrine portion of the organ [10] , [11] , [12] . Here we report how we utilized the wealth of biomedical information available today to form—and test—a hypothesis about the role of the primary cilium in pancreatic β-cell function. Although it is unclear whether diabetes is a secondary effect related to the truncal obesity phenotype of some ciliopathies, recent evidence suggests that in ALMS the diabetic phenotype might not be directly linked to body weight [6] . In patients with autosomal dominant polycystic kidney disease (ADPKD), a non-syndromic ciliopathy that does not present with truncal obesity, several parameters of β-cell function are reduced in comparison to controls [13] . A recent study shows a switch in glucose utilization to higher lactate production in murine Pkd1 −/− renal cells and kidney cells from ADPKD patients thus supporting a role for ciliary components in cellular glucose metabolism [14] . In addition, we observed that as many as two-thirds of the T2DM susceptibility genes have entries in the ciliary proteome database (see ref. 15 ), suggesting a direct relationship between ciliary dysfunction and T2DM susceptibility. In our study, we investigated the role of primary cilia in islet function and glucose homeostasis. To date, the majority of T2DM risk alleles are implicated with insulin secretion rather than insulin sensitivity of peripheral tissues. Before onset of obesity, we observed impaired glucose handling in Bbs4 −/− mice concomitant with blunted acute insulin release upon a glucose challenge. In stimulated β-cells, insulin receptor (IR) is recruited to the primary cilium; when ciliary/basal body integrity is impaired, phospho-activation of downstream signalling nodes is impaired suggesting that ciliary localization of IR is necessary for signal transduction. In a rat model of diabetes, we observed a reduction of ciliated β-cells and misexpression of ciliary/basal body components. This implicates a role for the primary cilium in glucose homeostasis, insulin signalling and T2DM disease risk. Pre-diabetic phenotypes in a ciliopathy model To test for a role of cilia in diabetes, we examined a ciliopathy model for pre-diabetic phenotypes. At birth, Bardet-Biedl-Syndrome 4 ( Bbs4 ) mutant mice are runted compared with their wild-type littermates and manifest obesity later on [15] . Penetrance is dependent on sex and age of the animals both in this and another Bbs4 −/− mutant strain [16] . Generally, female mutants are more severely affected than age-matched male mutants. At 4–6 months of age, both sexes exhibit diabetic phenotypes including hyperglycemia and mild hyperinsulinemia [15] . Because we could not exclude a role for Bbs4 during pancreas development, we assessed pancreatic islet morphology in 4-week-old male mutant mice and wild-type littermates ( n =3, Fig. 1a,b ). In contrast to the orpk (Oak Ridge polycystic kidney) mouse, an Intraflagellar Transport 88 ( Ift88 ) hypomorph, which displays abnormal pancreatic development starting at the end of gestation [10] , we did not observe overt morphological abnormalities in Bbs4 −/− mice such as pancreatic cysts. Islet morphology was not altered ( Fig. 1a,b ) other than a slightly skewed islet size distribution towards larger islets ( Fig. 1c ). Although the average islet size is shifted (2,045 versus 2,359 μm 2 ), the range is similar in both mutants and wild-type littermates. There is no discernible difference in serum insulin levels, implicating that, overall, Bbs4 −/− pancreatic islets develop normally ( Fig. 1d ). We did not find evidence of insulin hypersecretion as was previously reported for dense core granule exocytosis in C. elegans [17] . Similarly, the total pancreatic insulin content in Bbs4 −/− mice (male, 7–9 weeks, n =4) is not different from that of age-matched controls ( n =4; Fig. 1e ). We challenged male Bbs4 −/− mice and age-matched wild-type controls (7–9 weeks, n =5) with intraperitoneal injections of glucose (2 g kg −1 body weight) and monitored blood glucose levels over a 2-h period. Bbs4 mutants showed significantly impaired glucose handling with a delay in glucose clearance compared with controls ( t =80 min, 25.7 mM versus 16.5 mM blood glucose, * P =0.049 ( t -test), Fig. 1f ). Importantly, there is no significant difference in body weight between mutant and wild-type mice at this age ( Fig. 1g ) and thus impaired glucose handling precedes obesity. Previous studies have found differential distribution of white adipose tissue in several BBS mouse models [18] and we cannot completely exclude an effect of visceral fat pads on glucose tolerance in our animals. Still, we decided to focus our attention on the ciliary role in insulin secretion and β-cell function. 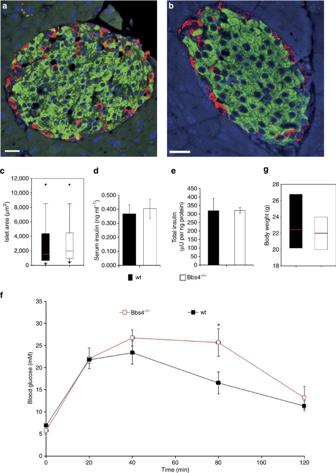Figure 1:Bbs4−/−mice manifest impaired glucose handling in the absence of morphological abnormalities in the pancreas. (a,b) Representative examples ofBbs4−/−(a) and littermate control (b) islets (n=3). Insulin is shown in green, glucagon in red, the nuclei are counterstained with 4,6-diamidino-2-phenylindole (DAPI; blue). Scale bars, 20 μm. (c) Islet size distribution is slightly skewed towards larger islets in 4-week-old maleBbs4−/−mice without clear differences in range (n=4). The red line demarks the median, the boxes the range from 25th to 75th percentile, the bars 10th and 90th percentile and the dots the 5th and 95th percentile of the size distribution. (d) Serum insulin levels are not significantly different between wt andBbs4−/−mice (4 weeks, male,n=4, error bars: standard deviation, st. dev.). (e) Total pancreatic insulin content is not statistically different between 7- and 9-week-oldBbs4−/−mice and littermate controls (n=4). (f) Glucose handling is significantly impaired inBbs4−/−mice (red) compared with littermate controls (black;n=5, 7–9 weeks;t=80 min, *P=0.0496 (t-test)). Error bars represent standard error, s.e.m. (g) At the age of glucose tolerance testing,Bbs4−/−and littermate controls have similar body weight. The boxes represent the 5th to 95th percentile and the red lines depict the median. Figure 1: Bbs4 −/− mice manifest impaired glucose handling in the absence of morphological abnormalities in the pancreas. ( a , b ) Representative examples of Bbs4 −/− ( a ) and littermate control ( b ) islets ( n =3). Insulin is shown in green, glucagon in red, the nuclei are counterstained with 4,6-diamidino-2-phenylindole (DAPI; blue). Scale bars, 20 μm. ( c ) Islet size distribution is slightly skewed towards larger islets in 4-week-old male Bbs4 −/− mice without clear differences in range ( n =4). The red line demarks the median, the boxes the range from 25th to 75th percentile, the bars 10th and 90th percentile and the dots the 5th and 95th percentile of the size distribution. ( d ) Serum insulin levels are not significantly different between wt and Bbs4 −/− mice (4 weeks, male, n =4, error bars: standard deviation, st. dev.). ( e ) Total pancreatic insulin content is not statistically different between 7- and 9-week-old Bbs4 −/− mice and littermate controls ( n =4). ( f ) Glucose handling is significantly impaired in Bbs4 −/− mice (red) compared with littermate controls (black; n =5, 7–9 weeks; t =80 min, * P =0.0496 ( t -test)). Error bars represent standard error, s.e.m. ( g ) At the age of glucose tolerance testing, Bbs4 −/− and littermate controls have similar body weight. The boxes represent the 5th to 95th percentile and the red lines depict the median. Full size image Disruption of basal body integrity impairs insulin secretion To examine the ciliary/basal body role in β-cell and islet function, we generated short hairpin RNA (shRNA) expression vectors targeting two different basal body genes namely Oral-facial-digital syndrome I ( Ofd1 ) and Bbs4 . Depletion of Ofd1 ultimately leads to loss of cilia (see ref. 19 and Supplementary Fig. 1C ), whereas loss of Bbs4 leaves cilia structurally intact but impairs cilia function [20] . Based on efficiency of knockdown as judged by mRNA levels and (in the case of Ofd1 ) reduced ciliation in MIN6m9 cells, a mouse insulinoma cell line, we selected one construct per gene for our experiments ( Supplementary Fig. 1 ). As a control, we used a scrambled RNA sequence in the same expression vector (shNC). For manipulation of primary islet cells, we shuttled the three different shRNA constructs (shOfd1, shBbs4, shNC) into a replication-deficient adenoviral vector and generated adenovirus for delivery of the expression vectors. This approach enabled us to target ciliary/basal body function in adult tissue homeostasis and we transduced islets from adult mice (C57B6/J) for our experiments. In our experience, the adenovirus penetrates deep into the islet albeit with reduced transduction towards the centre compared with the outer layers: we estimate the transduction efficiency at 40–45%. Overall, Ofd1 message was reduced by over 33% in islets treated with adenoviral shOfd1 and Bbs4 message by 45% in murine islets treated with adenoviral shBbs4 ( Supplementary Fig. 1D,E ). We recorded the insulin secretion profile in response to glucose and KCl ( Fig. 2a ): first phase insulin release is attenuated in both Ofd1 - and Bbs4 -depleted islets when compared with control islets ( t =58 min, ** P =0.001 (one-way analysis of variance (ANOVA))). The islets were responsive to other secretory stimuli including KCl, which is depolarizing the plasma membrane, opening the voltage-gated Ca 2+ -channels and increasing the cytoplasmic free Ca 2+ -concentration [Ca 2+ ] i (ref. 21 ). Although Ofd1 -depleted islets tended to have a slightly reduced secretory response to KCl, there was no statistical significance compared with scrambled controls ( t =98 min, P =0.775 (one way ANOVA)). To ensure that these effects were not due to off-target effects of the shRNA constructs targeting Bbs4 or Ofd1 , we designed a rescue experiment overexpressing human BBS4 in Bbs4 -depleted MIN6m9 cells ( Fig. 2b ). We incubated the cells in buffer containing 0.5 or 16.7 mM glucose in 5 min intervals. We then measured the insulin released into the supernatant and calculated the disposition index (DI) by normalizing the value for glucose-stimulated insulin release to the baseline value. The DI is an important clinical parameter of islet function [22] . We found a significant DI reduction in Bbs4 -depleted cells compared with controls ( Fig. 2b , 1.53±0.08 (s.e.m.) versus 2.39±0.18, n =6, P =0.024 (one way ANOVA)). Importantly, overexpression of myc-tagged human BBS4 also reduced the DI, similar to Bbs4 -depletion. To avoid confounding effects caused by the overexpression phenotype, we established a dose-response curve by overexpressing various amounts of mycBBS4 plasmid. The addition of 800 ng of plasmid to the Bbs4 -depleted cells increased the DI (1.88±0.13) but this increase was not statistically relevant ( n =5, P =0.861 (one way ANOVA)). Similarly, overexpression of 2,400 ng mycBBS4 yielded a statistically insignificant DI increase (1.90±0.08, n =4, P =0.871 (one way ANOVA)). By contrast, 1,600 ng mycBBS4 increased the DI significantly to levels indistinguishable from control cells (2.60±0.18, P =0.009 and P =0.994, respectively (one way ANOVA)). We therefore conclude that Bbs4 depletion leads to attenuated first phase insulin secretion. Because Ofd1 depletion yields a similar phenotype and both Ofd1 and Bbs4 localize to the basal body, we suggest that basal body/ciliary perturbation per se has this effect on biphasic insulin secretion. Notably, early in the course of T2DM, patients manifest a selective loss of glucose-stimulated first phase insulin release while maintaining the response to other secretagogues [23] . α- and δ-cells are also ciliated and we cannot exclude a role for primary cilia of other endocrine cells in the regulation of insulin or other islet hormones. However, as similar manipulations in MIN6m9 cells also resulted in a loss of first phase insulin release ( Fig. 2b and Supplementary Fig. 2A ), we suggest that the primary player might be the β-cell cilium. 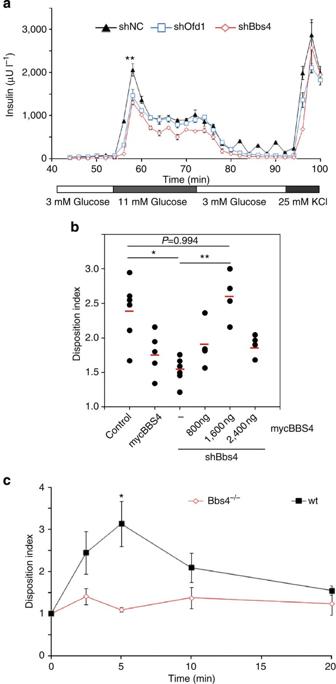Figure 2: First phase insulin release is blunted when basal bodies/cilia are disrupted. (a) Whole islets depleted of Ofd1(blue) or Bbs4 (red) have an attenuated first phase when stimulated with glucose but react normally to potassium chloride (t=58 min, **P=0.001 (one-way ANOVA), error bars: st. dev.). (b) Re-introduction of myc-taggedBbs4rescues the disposition index in shBbs4-treated cells.P(shNC versus shBbs4)=0.024;P(shBbs4 versus shBbs4+1,600 ng mycBBS4)=0.000;P(shNC versus shBbs4+1,600 ng mycBBS4)=0.994 (one-way ANOVA). (c) The acute insulin response to glucose in Bbs4−/−mice (red) is significantly attenuated compared with age- and weight-matched controls (black;n=4,t=5 min, *P=0.039, error bars: s.e.m.). Figure 2: First phase insulin release is blunted when basal bodies/cilia are disrupted. ( a ) Whole islets depleted of Ofd1(blue) or Bbs4 (red) have an attenuated first phase when stimulated with glucose but react normally to potassium chloride ( t =58 min, ** P =0.001 (one-way ANOVA), error bars: st. dev.). ( b ) Re-introduction of myc-tagged Bbs4 rescues the disposition index in shBbs4-treated cells. P (shNC versus shBbs4)=0.024; P (shBbs4 versus shBbs4+1,600 ng mycBBS4)=0.000; P (shNC versus shBbs4+1,600 ng mycBBS4)=0.994 (one-way ANOVA). ( c ) The acute insulin response to glucose in Bbs4 −/− mice (red) is significantly attenuated compared with age- and weight-matched controls (black; n =4, t =5 min, * P =0.039, error bars: s.e.m.). Full size image To probe for physiological relevance for our in vitro findings, we sampled serum insulin over the first 20 min of an intraperitoneal glucose challenge (2 g kg −1 ). We found that the DI of stimulated serum insulin levels normalized to fasted serum insulin was significantly reduced in Bbs4 mutants compared with that of age-matched wild-type controls ( Fig. 2c , t=5 min, 1.1-fold versus 3.1-fold stimulation over baseline ( t =0 min, * P =0.039 ( t -test)). We did not observe a significant difference in absolute serum insulin levels, in part because of a high variability of fasting serum insulin levels among controls ( Supplementary Fig. 2B ). The fasted serum insulin levels in Bbs4 −/− mice tended to be higher than in controls, although the difference was not significant. Because various glucose transporters are also listed in the ciliaproteome database, we tested for glucose uptake in cells with and without Bbs4 or Ofd1 but did not observe a difference between groups (data not shown). Moreover, the β-cell cilium might play a central role in cellular metabolism; therefore, we tested for changes in cellular energetics on a Seahorse flux analyzer. Under the chosen conditions, we did not observe differences in oxygen consumption, suggesting that overall β-cell metabolism in response to glucose is unaffected by loss of ciliary function ( Fig. 3a ). In vitro and in vivo data strongly point to a ciliary involvement in first phase insulin release. 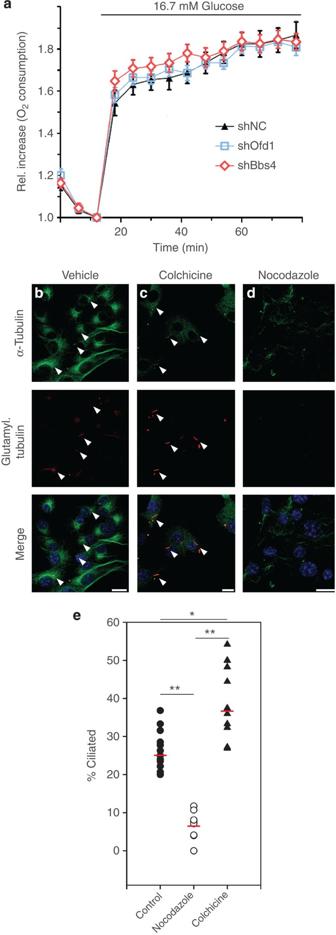Figure 3: The effect is independent of glucose metabolism and likely cilia specific. (a) In MIN6m9 cells treated with adenoviral constructs, no difference in oxygen consumption after glucose stimulation (normalized to baseline) in the presence (black) or absence of Ofd1 (blue) or Bbs4 (red) was observed. OCR was determined on a Seahorse flux analyzer. (b–d) Colchicine treatment leaves the ciliary axoneme (glutamylated tubulin, red) of MIN6 cells intact. Treatment with nocodazole disrupts the microtubular network (d; α-tubulin, green) and the ciliary axoneme, whereas colchicine dissolves the microtubular network but leaves the ciliary axoneme intact (c). Nuclei are depicted in blue (4,6-diamidino-2-phenylindole, DAPI). Shown are maximum projections of representative confocal stacks. Scale bars, 5 μm. Arrowheads highlight the ciliary axoneme. (e) Percentage of ciliated MIN6m9 cells treated with vehicle (solid circles), nocodazole (open circles) or colchicine (solid triangles). Red bars depict the mean. **P(vehicle versus nocodazole)<0.001; **P(nocodazole versus colchicine)<0.001 (one-way ANOVA). *P<0.01. The observations were made on three different occasions,n(vehicle)=n(control)=12,n(nocodazole)=9 (totalNof cells observed: 240 (vehicle), 241 (nocodazole), 314 (colchicine)). Figure 3: The effect is independent of glucose metabolism and likely cilia specific. ( a ) In MIN6m9 cells treated with adenoviral constructs, no difference in oxygen consumption after glucose stimulation (normalized to baseline) in the presence (black) or absence of Ofd1 (blue) or Bbs4 (red) was observed. OCR was determined on a Seahorse flux analyzer. ( b – d ) Colchicine treatment leaves the ciliary axoneme (glutamylated tubulin, red) of MIN6 cells intact. Treatment with nocodazole disrupts the microtubular network ( d ; α-tubulin, green) and the ciliary axoneme, whereas colchicine dissolves the microtubular network but leaves the ciliary axoneme intact ( c ). Nuclei are depicted in blue (4,6-diamidino-2-phenylindole, DAPI). Shown are maximum projections of representative confocal stacks. Scale bars, 5 μm. Arrowheads highlight the ciliary axoneme. ( e ) Percentage of ciliated MIN6m9 cells treated with vehicle (solid circles), nocodazole (open circles) or colchicine (solid triangles). Red bars depict the mean. ** P (vehicle versus nocodazole)<0.001; ** P (nocodazole versus colchicine)<0.001 (one-way ANOVA). * P <0.01. The observations were made on three different occasions, n (vehicle)= n (control)=12, n (nocodazole)=9 (total N of cells observed: 240 (vehicle), 241 (nocodazole), 314 (colchicine)). Full size image The effect on insulin secretion is likely cilia specific Suppression of two independent genes, Ofd1 and Bbs4 (both encode basal body proteins), results in a loss of first phase insulin secretion, pointing to a role for basal body/ciliary integrity in insulin release. However, because both proteins might also have non-ciliary functions, we could not fully exclude that the phenotype is not cilia specific; for example, BBS4 depletion has effects on organization of the microtubular (MT) skeleton [24] . Early investigations into the mechanism of insulin release had revealed that the disruption of the MT network resulted in loss of insulin release, indicating that MT transport is essential for insulin secretion [25] . In contrast to MT effectors like nocodazole, treatment with colchicine abolished second phase insulin release but rendered the first phase intact [26] , [27] , [28] , [29] . We sought to confirm these findings and found a loss of second but not first phase insulin release for colchicine-treated MIN6m9 cells and isolated murine islets, whereas there was no insulin released in the case of treatment with nocodazole (data not shown). In tetrahymena pyriformis , it has been shown that colchicine does not disrupt existing ciliary axonemes [30] and we found previously that vinblastine, a drug with a similar mechanism of action, left the ciliary axoneme of human embryonic kidney cells (HEK293T) intact [31] . At the same time, nocodazole in moderate to high concentrations has been shown to disrupt the ciliary axoneme along with the MT network [32] , [33] . In line with these observations, nocodazole dissolved the MT skeleton including the ciliary axoneme of the MIN6m9 β-cell line, whereas colchicine did not disassemble the ciliary axoneme ( Fig. 3b–e ). When treated with vehicle, 26.7±1.5% (s.e.m.) of cells were ciliated ( Fig. 3b,e ). Nocodazole treatment reduced the number of ciliated cells to 6.7±1.4% ( P <0.001, Fig. 3d,e ), whereas we observed an increase in ciliated cells upon colchicine treatment (38±3.0%, P =0.006 (one-way ANOVA), Fig. 3c,e ). We cannot exclude an effect of colchicine on ciliogenesis, although a parsimonious explanation might be the improved visibility of ciliary axonemes because of the absence of other acetylated MT structures that otherwise mask the axonemes. These findings not only corroborate our previous results and strongly implicate a specific role for the cilium in first phase insulin release; they also offer an explanation for an almost 40-year-old observation, the differential effect of colchicine and nocodazole on insulin secretion [26] , [27] , [28] . IR is recruited to the β-cell cilium Mice lacking functional IR in β-cells (β-cell-specific Insulin Receptor Knockout mice, βIRKO) show several phenotypes characteristic of T2DM susceptibility. Notably, they have a compromised first phase insulin release in response to a glucose challenge [34] . Over time, 25% of βIRKO mice become diabetic as judged by an intraperitoneal glucose tolerance test; however, both diabetic and non-diabetic βIRKO mice manifest blunted acute insulin secretion when challenged with intra-peritoneal glucose injections [35] . Bbs4 −/− mice manifest a similar phenotype when challenged with glucose and this is phenocopied by disruption of either Bbs4 or Ofd1 in intact islets and a β-cell line. Therefore, we speculated that IR localizes to the primary cilium and that this localization is necessary for proper function of the IR. In stimulated MIN6m9 cells (5 mU ml −1 insulin, 3 min), IR localizes to the primary cilium as well as other cellular compartments including plasma membrane and vesicles ( Fig. 4a ). We also found IR on cilia of stimulated human primary β-cells ( Fig. 4b ). Because β-cells express two isoforms of IR that differ in the presence (IR B) or absence (IR A) of exon 11 of the Insr gene, we used a selective antibody raised against IR B to probe for a preferential recruitment of one isoform over the other. We found no recruitment of IR B to the cilium in response to insulin stimulation ( Fig. 4c ). Because of a lack of IR A-selective antibodies, we next expressed epitope-tagged IR A and IR B , respectively. In unstimulated cells, we did not observe IR A on the cilium, whereas it was still present in other cellular compartments ( Fig. 4d ). In stimulated cells, we found specific ciliary recruitment of IR A ( Fig. 4e ), whereas we did not find IR B on cilia regardless of insulin stimulation ( Fig. 4f ). We found IR A on 2 out of 31 compared with 16 out of 34 cilia in unstimulated versus stimulated cells in a blind study ( n >100 cells, three independent experiments, P =0.002 (Fisher exact test)). We repeated our experiments with another ciliary marker, glutamylated (de-tyrosinated) α-tubulin and also observed ciliary recruitment for IR A in the presence of insulin only ( Fig. 4g,h ). As a control for specificity of recruitment, we expressed epitope-tagged IGF1 Receptor ( IGF1R ) in the same β-cell line. Ciliary IGF1R localization has been observed in differentiating adipocytes [36] ; under our experimental conditions, we did not observe IGF1R localization to the cilium (data not shown). Although there are numerous examples of ciliary membrane components that—when heterologously expressed—still localize to the ciliary membrane, our observation implies that, in the MIN6m9 cell line, sorting to the ciliary membrane compartment is tightly controlled even when potential ciliary components are overexpressed. 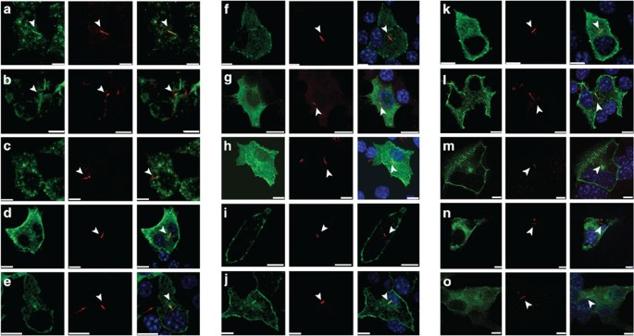Figure 4: IR is recruited to the primary cilium of stimulated β-cells. Cilia are shown in red; ina–f,i–k, we used a mixture of anti-acetylated α-tubulin and anti-γ-tubulin antibodies, ing–h,l, we used anti-glutamylated α-tubulin antibody and inm–o, we used anti-Arl13b antibody to visualize the primary cilium. (a,b) Insulin receptor (green) localizes to the primary cilium of insulin-stimulated MIN6m9 (a) and human primary β-cells (b; 5 mU ml−1, 3 min). The arrowhead points to a cilium of a β-cell (insulin staining not shown), in b is the ciliated adjacent cell not a β-cell. (c) IR B (green) is not recruited to the ciliary compartment of insulin-stimulated cells. (d) In unstimulated MIN6m9 cells, epitope-tagged IR A (green) does not localize to the primary cilium (red) over the course of observation. (e) Epitope-tagged IR A is recruited to the primary cilium in insulin-stimulated cells (5 mU ml−1, 3 min). (f) Epitope-tagged IR B does not localize to cilia of insulin-stimulated cells. (g) In unstimulated MIN6m9 cells, IR A does not localize to the cilium (glutamyl. tubulin). (h) After stimulation with 5 mU ml−1insulin for 3 min, IR A is recruited to the primary cilium (glutamyl. tubulin). (i) Epitope-tagged kinase-dead IR A does not localize to cilia of insulin-stimulated cells. (j) Epitope-tagged constitutively active IR A (V938D) localizes to the ciliary membrane even in the absence of insulin. (k) Epitope-tagged constitutively active IR B (V950D) does not localize to the ciliary membrane in the absence or presence of insulin. (l) Constitutively active IR A V950D mutant localizes to the cilium (red, glutamyl. tubulin) of unstimulated MIN6m9 cells. (m–o) Using Arl13b as ciliary marker, we also observed IR A (m) on the cilium of insulin-stimulated MIN6m9 cells, but not on that of unstimulated cells (n). (o) In stimulated MIN6m9 cells, IR B does not localize to the cilium. Ina–h,j–o, nuclei are shown in blue (4,6-diamidino-2-phenylindole, DAPI). With the exception of b, cells shown are MIN6m9 cells. Shown are single images, scale bars, 5 μm. Figure 4: IR is recruited to the primary cilium of stimulated β-cells. Cilia are shown in red; in a – f , i – k , we used a mixture of anti-acetylated α-tubulin and anti-γ-tubulin antibodies, in g – h , l , we used anti-glutamylated α-tubulin antibody and in m – o , we used anti-Arl13b antibody to visualize the primary cilium. ( a , b ) Insulin receptor (green) localizes to the primary cilium of insulin-stimulated MIN6m9 ( a ) and human primary β-cells ( b ; 5 mU ml −1 , 3 min). The arrowhead points to a cilium of a β-cell (insulin staining not shown), in b is the ciliated adjacent cell not a β-cell. ( c ) IR B (green) is not recruited to the ciliary compartment of insulin-stimulated cells. ( d ) In unstimulated MIN6m9 cells, epitope-tagged IR A (green) does not localize to the primary cilium (red) over the course of observation. ( e ) Epitope-tagged IR A is recruited to the primary cilium in insulin-stimulated cells (5 mU ml −1 , 3 min). ( f ) Epitope-tagged IR B does not localize to cilia of insulin-stimulated cells. ( g ) In unstimulated MIN6m9 cells, IR A does not localize to the cilium (glutamyl. tubulin). ( h ) After stimulation with 5 mU ml −1 insulin for 3 min, IR A is recruited to the primary cilium (glutamyl. tubulin). ( i ) Epitope-tagged kinase-dead IR A does not localize to cilia of insulin-stimulated cells. ( j ) Epitope-tagged constitutively active IR A (V938D) localizes to the ciliary membrane even in the absence of insulin. ( k ) Epitope-tagged constitutively active IR B (V950D) does not localize to the ciliary membrane in the absence or presence of insulin. ( l ) Constitutively active IR A V950D mutant localizes to the cilium (red, glutamyl. tubulin) of unstimulated MIN6m9 cells. ( m – o ) Using Arl13b as ciliary marker, we also observed IR A ( m ) on the cilium of insulin-stimulated MIN6m9 cells, but not on that of unstimulated cells ( n ). ( o ) In stimulated MIN6m9 cells, IR B does not localize to the cilium. In a – h , j – o , nuclei are shown in blue (4,6-diamidino-2-phenylindole, DAPI). With the exception of b, cells shown are MIN6m9 cells. Shown are single images, scale bars, 5 μm. Full size image Expression of a kinase-dead IR A construct showed no ciliary localization irrespective of insulin stimulation ( Fig. 4i ; 1/20 versus 0/20 positive cilia in unstimulated/stimulated cells; n >80 cells, three independent experiments), indicating that tyrosine kinase activity plays a role in the recruitment process. A constitutively active IR A mutant (V950D IR A) [37] localizes to the ciliary membrane even in unstimulated MIN6m9 cells, whereas the corresponding IR B mutant (V950D IR B) does not ( Fig. 4j,k ; V950D IR A was observed on 14/15 cilia versus V950D IR B was observed on 0/16 cilia; P =0.0005 (Fisher exact test); n >60 cells, three independent experiments). Using alternate ciliary marker glutamylated tubulin, we also observed IR A V950D ( Fig. 4l ), but not IR B V950D on the cilium. Another ciliary marker, Arl13b, also revealed ciliary recruitment of IR A but not IR B in an insulin-stimulated, but not unstimulated β-cell line ( Fig. 4m–o ). We confirmed activity of IR V950D mutants by quantification of tyrosine phosphorylation at Y972 in immunoprecipitated IR. No significant difference in phosphorylation was observed between insulin-stimulated wild-type IR and unstimulated V950D mutants ( Supplementary Fig. 3 ). Our observation suggests that activation of IR A is necessary and sufficient for ciliary localization. Ciliary IR localization is necessary for insulin signalling Specific localization often points to the site of action of the protein. If ciliary localization is indeed necessary for IR signalling activity, we should expect downstream components of the IR signalling cascade to be affected with basal body/ciliary impairment. We have shown that basal body/ciliary disruption phenocopies the loss of IR activity in stimulated β-cells and islets with respect to insulin secretion. Insulin signalling is transmitted through a highly complex network of essential mediators and modifiers of the signal. Three nodes have been identified for insulin signalling: the family of insulin receptor substrate proteins (IRS), the different subunits of phosphatidylinositol-3-kinase (PI3K) and the serine/threonine protein kinase Akt/PKB (protein kinase B) family downstream of PI3K [38] . The p85 and p55 splice isoforms of the Pi3kr1 regulatory subunit of PI3K are phosphorylated at residues Tyr458 or Tyr199, respectively, in response to upstream signal activation [39] . In MIN6m9 cells, we found the p55 splice isoform to be the main target of insulin-stimulated tyrosine phosphorylation. In insulin-stimulated, Bbs4 -depleted cells, we observed a robust reduction in phospho-p55 (pTyr199) by 80–90% compared with stimulated control cells ( n =3, Fig. 5a and Supplementary Fig. 6 ; normalized to loading control γ-tubulin). Similarly, reduced phospho-p55 levels were observed in Ofd1 -depleted cells. 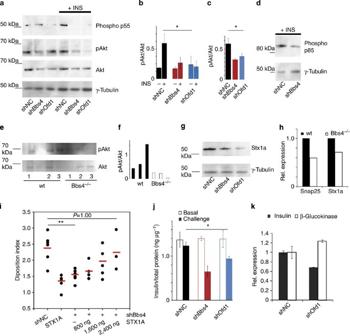Figure 5: Ciliary/basal body disruption impairs insulin receptor-mediated signalling. (a) Immunoblotting of basal and insulin-stimulated levels of phosphorylated p55 (pTyr199), phospho-Akt (pSer473), pan-Akt and γ-tubulin in lysates of MIN6m9 cells transduced with adenovirus targetingOfd1(shOfd1),Bbs4(shBbs4) alongside scrambled RNA (shNC). (b) pSer473 Akt to pan-Akt ratio in the presence or absence ofBbs4andOfd1in basal (INS-) and stimulated (INS +) MIN6m9 cells (*P=0.035 for insulin-stimulated levels, one-way ANOVA). (c) pSer472 Akt to pan-Akt ratio in insulin-stimulatedBbs4- orOfd1-depleted murine islets (*P=0.042, one-way ANOVA). (d) Phosphorylated p85 (pTyr458) in insulin-stimulated murine islets transduced with adenovirus targetingBbs4and scrambled RNA control. (e) pSer473 Akt is reduced in islets from threeBbs4−/−animals compared with wild-type controls. (f) Phospho Akt/Akt ratio forBbs4−/−and wild-type animals. (g) Syntaxin1A levels are reduced inOfd1- orBbs4-depleted islets compared with controls. (h) Relative expression levels ofSnap25andStx1aare reduced in islets ofBbs4−/−animals compared with wild-type controls (RNA pooled from three animals each). (i) Re-introduction ofSTX1A- intoBbs4-depleted MIN6m9 cells partially restores the disposition index. **P(control versus shBbs4)=0.007,P(shNC versus shBbs4+1,600 ngSTX1A)=0.417,P(shNC versus shBbs4+2,400 ngSTX1A)=1.00, one-way ANOVA (Tukey’s). Red bars indicate the mean. (j) Under basal conditions (open bars), insulin content is similar to controls (shNC, black) in MIN6m9 cells treated with adenoviral shOfd1 (blue) or shBbs4 (red). After 30 min of 16.7 mM glucose and another 15 min 25 mM KCl, the total insulin content (solid bars) in Ofd1- (blue) or Bbs4- (red) depleted cells is significantly decreased compared with control cells (n=8,P=0.002, (one-way ANOVA)). (k) One hour after insulin stimulation,InsmRNA is reduced by up to 40%, whereasβGckmRNA is slightly but not significantly upregulated inOfd1-depleted MIN6m9cells (n=3). Error bars: st. dev. Figure 5: Ciliary/basal body disruption impairs insulin receptor-mediated signalling. ( a ) Immunoblotting of basal and insulin-stimulated levels of phosphorylated p55 (pTyr199), phospho-Akt (pSer473), pan-Akt and γ-tubulin in lysates of MIN6m9 cells transduced with adenovirus targeting Ofd1 (shOfd1), Bbs4 (shBbs4) alongside scrambled RNA (shNC). ( b ) pSer473 Akt to pan-Akt ratio in the presence or absence of Bbs4 and Ofd1 in basal (INS-) and stimulated (INS +) MIN6m9 cells (* P =0.035 for insulin-stimulated levels, one-way ANOVA). ( c ) pSer472 Akt to pan-Akt ratio in insulin-stimulated Bbs4 - or Ofd1 -depleted murine islets (* P =0.042, one-way ANOVA). ( d ) Phosphorylated p85 (pTyr458) in insulin-stimulated murine islets transduced with adenovirus targeting Bbs4 and scrambled RNA control. ( e ) pSer473 Akt is reduced in islets from three Bbs4 −/− animals compared with wild-type controls. ( f ) Phospho Akt/Akt ratio for Bbs4 −/− and wild-type animals. ( g ) Syntaxin1A levels are reduced in Ofd1 - or Bbs4 -depleted islets compared with controls. ( h ) Relative expression levels of Snap25 and Stx1a are reduced in islets of Bbs4 −/− animals compared with wild-type controls (RNA pooled from three animals each). ( i ) Re-introduction of STX1A - into Bbs4 -depleted MIN6m9 cells partially restores the disposition index. ** P (control versus shBbs4)=0.007, P (shNC versus shBbs4+1,600 ng STX1A )=0.417, P (shNC versus shBbs4+2,400 ng STX1A )=1.00, one-way ANOVA (Tukey’s). Red bars indicate the mean. ( j ) Under basal conditions (open bars), insulin content is similar to controls (shNC, black) in MIN6m9 cells treated with adenoviral shOfd1 (blue) or shBbs4 (red). After 30 min of 16.7 mM glucose and another 15 min 25 mM KCl, the total insulin content (solid bars) in Ofd1- (blue) or Bbs4- (red) depleted cells is significantly decreased compared with control cells ( n =8, P =0.002, (one-way ANOVA)). ( k ) One hour after insulin stimulation, Ins mRNA is reduced by up to 40%, whereas βGck mRNA is slightly but not significantly upregulated in Ofd1 -depleted MIN6m9cells ( n =3). Error bars: st. dev. Full size image Among the residues that are phosphorylated over the course of Akt kinase activation is Ser473 in the C-terminal portion of the protein [40] , [41] . Depletion of Ofd1 or Bbs4 reproducibly results in reduced phospho-Akt (pSer473) after insulin stimulation (5 mU ml −1 , 15 min) in MIN6m9 cells ( Fig. 5a ). To better quantify the size of the effect, we used an ELISA-based system to determine the phospho-Akt (pSer473)/Akt ratio and found that insulin-dependent Ser473 Akt phosphorylation is almost completely abolished in Bbs4 - or Ofd1 -depleted MIN6m9 cells ( P =0.035 (one-way ANOVA), Fig. 5b ). We also probed for Akt activation in primary cells, specifically in intact islets that were transduced with adenovirus targeting either Bbs4 or Ofd1 , respectively, along with scrambled RNA as a control ( Fig. 5c ). In insulin-stimulated Bbs4 - or Ofd1 -depleted islets, we found the pSer473 Akt/Akt ratio reduced by 46% and 34%, respectively, consistent with our findings in MIN6m9 cells ( n =3, P =0.042 (one-way ANOVA)). The Pik3r1 splice isoform that is tyrosine-phosphorylated in response to insulin is p85. Phospho-p85 (pTyr458) decreased by ~60% in Bbs4 -depleted islets ( Fig. 5d , n =3, normalized to loading control γ-tubulin). Similarly, we found a reduction in pSer473 Akt in islets from three different Bbs4 −/− mice compared with wild-type littermates ( Fig. 5e,f ). Pik3r2 −/− mice with a β-cell-specific deletion of Pik3r1 manifest marked glucose intolerance, at least partially due to a loss of acute insulin secretion when challenged with intraperitoneal glucose injections [42] . Islets of these animals express significantly less exocytotic proteins involved in SNARE (soluble N -ethylmaleimide attachment receptor) complex formation because of impaired FoxO1 transcriptional activity [42] . One of these proteins regulated by FoxO1, Syntaxin1A, interacts with the α1D subunit of the L-type voltage-gated Ca 2+ channel [43] and is implicated in SNARE formation and insulin release [44] . An orthologue in C. elegans is regulated by daf-19 , a transcription factor that is expressed in all ciliated sensory neurons [45] , [46] . We found Syntaxin1A (Stx1a) protein levels reduced by 25–30% in Bbs4 -depleted islets and by 30–40% in Ofd1 -depleted islets ( Fig. 4g , n =3, normalized to loading control γ-tubulin). In Bbs4 −/− islets, we observed a reduction of Snap25 and Stx1A mRNA levels by 41% and 29%, respectively ( Fig. 5h ). Because pre-assembled Snap25/Syntaxin1A complexes have been implicated in first phase insulin release [44] , it is possible that reduction of one or more SNARE subunits changes the steady-state equilibrium of at least two preparatory configurations of SNARE complexes. To test a role for Stx1a reduction in the observed loss of first phase insulin release, we attempted to rescue insulin release by overexpression of STX1A in Bbs4 -depleted MIN6m9 cells ( Fig. 5i ). Overexpression of STX1A deregulates insulin release, increasing basal secretion to a point when added glucose does not increase insulin secretion any further; this unresponsiveness to glucose is reflected in a decreased DI (1.31±0.11 versus 2.39±0.18 for control, n =5, P <0.001, one-way ANOVA). We established a dose-response curve by overexpressing various amounts of STX1A in Bbs4 -depleted cells ( Fig. 5i ). Although Bbs4 -depleted cells have a significantly reduced DI (1.53±0.08), introduction of moderate to high amounts of STX1A increases the DI to levels that are no longer statistically different from controls (shBbs4+1,600 ng STX1A , DI=1.92±0.21, n =5, P =0.417, and shBbs4+2,400 ng STX1A , DI=2.27±0.36, n =3, P =1.00 (one-way ANOVA)). Our data suggest that reduced Stx1a protein levels are partially responsible for the attenuation of first phase insulin release. We did not achieve a full rescue of the observed phenotype, which could be explained by reduced levels of Snap25 expression. Overall, our experiments indicate that loss of IR signalling in β-cells leads to loss of first phase insulin secretion via a loss of PI3K/FoxO1-regulated transcription of SNARE components Stx1a and Snap25 . MIN6m9 cells depleted of Ofd1 or Bbs4, respectively, contained overall less insulin than those treated with scrambled RNA immediately after a glucose and KCl challenge ( n =3, P =0.005 (one-way ANOVA), Supplementary Fig. 4 ). We have previously reported that IR A specifically regulates Insulin ( Ins ) transcription, whereas IR B regulates transcription of β-cell-specific glucokinase ( βGck ) in response to insulin stimulation [47] . In contrast, Bbs4 −/− mice have a normal pancreatic insulin content ( Fig. 1e ) and, although the pancreatic insulin content in βIRKO mice is reduced, this observation has been linked to reduced β-cell mass [35] . We argue that IR A-dependent transcriptional regulation of Ins will be particularly active while insulin is secreted in response to glucose or other secretagogues. Therefore, we determined the insulin content in Bbs4 - or Ofd1 -depleted MIN6m9 cells under basal conditions (0.5 mM glucose) and after treatment with 16.7 mM glucose for 30 min, followed by a potassium challenge (25 mM KCl) for another 15 min ( Fig. 5j , n =8). We observed no difference in insulin content (normalized to total protein) between control and Bbs4 / Ofd1 -depleted cells under basal conditions. However, after a glucose challenge and membrane depolarization, we observed reduced amounts of insulin of Bbs4 -/ Ofd1 -depleted cells compared with controls. We suggest that reduction in insulin content strongly implicates a requirement of ciliary localization for IR A signalling activity. The effect on IR B signalling function, however, remained unclear. To address this branch of the insulin signalling pathway, we suppressed ciliogenesis by disrupting Ofd1 -message in MIN6m9 cells and monitored Ins and βGck expression after insulin stimulation. Quantitative real-time PCR revealed that Ins message was reduced in Ofd1 -depleted cells, whereas βGck message was not significantly changed ( n =3, Fig. 5k ), further supporting the specific role for primary β-cell cilia in IR A-mediated insulin signalling. The ciliary recruitment of IR A but not IR B supports our earlier finding of distinct signalling activities [47] and spatial segregation [48] of the two isoforms. Also in line with earlier observations is the robust loss of p85/p55 activation in cells with compromised basal body/ciliary integrity; of note, we have described a preferential co-distribution of IR A with Class Ia PI3K [49] . It remains to be seen if there is a role for basal body/ciliary proteins in other target tissues of insulin action such as muscle. Ciliary phenotypes in a T2DM rat model We have found that ciliary/basal body defects lead to pre-diabetic phenotypes in vitro and in vivo , but to establish a link between primary cilia and diabetes, we tested for ciliary dysfunction in diabetic Goto-Kakizaki (GK) rats [50] , [51] . GK rats from the Stockholm colony manifest a marked glucose intolerance with hyperglycemia, mainly due to impaired glucose-stimulated insulin secretion. At the age studied (2–3 months), β-cell density and relative volume of islet endocrine cells are similar to those of age-matched control Wistar rats [50] . At the time of the experiment, blood glucose levels were elevated ( n =10, 7.2 to 10.2 mM) compared with Wistar controls ( n =12, 5.1–6.4 mM). We removed pancreata from three GK rats and three age-matched Wistar rats and quantified number and length of β-cell cilia. To minimize bias, the investigator was blinded to the strain of animals when taking confocal images and the file names of the image series were subsequently changed to add an additional blindfold to the image analysis process. We defined the region of interest (ROI) based on insulin staining to select for β-cells ( Fig. 6a–d ). Because nerve fibres also contain the ciliary marker acetylated α-tubulin ( Supplementary Fig. 5A–F ), we automatically excluded all objects greater than 1 μm 3 in volume or 15 μm in length. The remaining objects were visually inspected and either included or excluded from the final cilia count. In total, we analysed ten islets each from two non-consecutive sections for each animal ( n =3 GK, n =3 Wistar, Fig. 6a–d ). We found significantly less ciliated β-cells in individual GK rats compared with Wistar controls ( P =0.000 (one-way ANOVA), Fig. 6e ). Pooling the data per strain, we found an overall approximately threefold reduction of ciliated β-cells (60 islets per animal strain, P =0.000 ( t -test), Fig. 6f ). The length of cilia was similar in both GK and Wistar rats ( Fig. 6g ). Quantitative real-time PCR studies revealed misregulation of several ciliary/basal body genes in isolated pancreatic islets from GK compared with Wistar rats ( n =6, Fig. 6h ). Pericentriolar material 1 (Pcm1), a centriolar and basal body protein, is approximately threefold upregulated in GK islets as has been shown previously [52] . Similarly, Bbs4 and Ift88, a component of intraflagellar transport complex B, are ~2.5-fold upregulated ( Fig. 6h ). We also found increased Pcm1 and Kif3a protein levels in GK islets compared with Wistar control islets ( n =3, Fig. 6i and Supplementary Fig. 7 ). In addition and as reported previously [50] , we observed a reduction of Stx1a levels in GK rats compared with Wistar controls. The seeming discrepancy between loss of function and increased expression levels could indicate a compensatory mechanism in reaction to impairment of ciliary/basal body integrity. Importantly, GK rat islets have reduced levels of exocytotic proteins including SNARE subunit Syntaxin1A [52] . Evidence of ciliary dysfunction in islets from a diabetic animal model strongly suggests a role for the β-cell cilium in T2DM susceptibility. 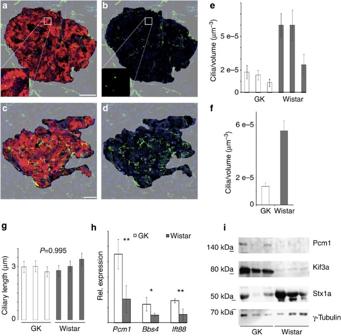Figure 6: Ciliary defects in Goto-Kakizaki rats. (a–d) Examples of image analysis on Wistar (a,b) and GK rats (c,d). β-Cells were identified based on insulin staining (red). We used anti-acetylated α-tubulin to visualize cilia. Insulin-negative tissue was masked (shown in grey) and the analysis of the green channel was limited to the β-cell area. Examples of cilia are emphasized in the enlarged insets corresponding to the areas highlighted by the white boxes. Scale bars, 20 μm. (e,f) The number of ciliated β-cells is reduced in GK compared with age-matched Wistar rats. (e) Average ratio of cilia to β-cell volume in three individual animals per strain (n=20 per group,P=0.000 (one-way ANOVA) error bars: s.e.m.). (f) Ratio of cilia number to β-cell volume in pooled islets of each strain (n=60,P=0.000, error bars: s.e.m.). (g) Ciliary length is similar in GK and Wistar rats (20 islets per animal were analysed, (one-way ANOVA) error bars: s.e.m.). (h) Basal body and ciliary genes are misregulated in GK compared with Wistar controls (n=6, *P=0.021, **P<0.01 (one-way ANOVA), error bars: st. dev.).Pcm1,Bbs4andIft88message were normalized to the 18S ribosomal subunit. (i) Pcm1 and Kif3a protein levels are increased, whereas Stx1a levels are decreased in GK islets compared with Wistar controls (n=3, loading control: γ-tubulin). Figure 6: Ciliary defects in Goto-Kakizaki rats. ( a – d ) Examples of image analysis on Wistar ( a , b ) and GK rats ( c , d ). β-Cells were identified based on insulin staining (red). We used anti-acetylated α-tubulin to visualize cilia. Insulin-negative tissue was masked (shown in grey) and the analysis of the green channel was limited to the β-cell area. Examples of cilia are emphasized in the enlarged insets corresponding to the areas highlighted by the white boxes. Scale bars, 20 μm. ( e , f ) The number of ciliated β-cells is reduced in GK compared with age-matched Wistar rats. ( e ) Average ratio of cilia to β-cell volume in three individual animals per strain ( n =20 per group, P =0.000 (one-way ANOVA) error bars: s.e.m.). ( f ) Ratio of cilia number to β-cell volume in pooled islets of each strain ( n =60, P =0.000, error bars: s.e.m.). ( g ) Ciliary length is similar in GK and Wistar rats (20 islets per animal were analysed, (one-way ANOVA) error bars: s.e.m.). ( h ) Basal body and ciliary genes are misregulated in GK compared with Wistar controls ( n =6, * P =0.021, ** P <0.01 (one-way ANOVA), error bars: st. dev.). Pcm1 , Bbs4 and Ift88 message were normalized to the 18S ribosomal subunit. ( i ) Pcm1 and Kif3a protein levels are increased, whereas Stx1a levels are decreased in GK islets compared with Wistar controls ( n =3, loading control: γ-tubulin). Full size image In this study, we propose a role for the primary cilium in insulin secretion, insulin signalling and glucose metabolism. If, indeed, ciliary dysfunction contributes to an individual’s risk to develop T2DM, four a priori statements should be true: First, there should be phenotypic overlap between ciliopathies and susceptibility to diabetes mellitus . Impaired glucose tolerance or even T2DM is a common symptom in ciliopathies such as BBS or ALMS [5] , [6] and ADPKD patients also show evidence of abnormal glucose handling [13] . Moreover, male Bbs4 −/− mice manifest impaired glucose handling compared with age- and weight-matched controls before the onset of obesity, implicating a role for cilia in glucose metabolism. Second, ciliary/basal body perturbation should lead to insulin resistance and/or β-cell dysfunction, the main metabolic variables in T2DM. Disruption of basal body/ciliary integrity by suppression of two independent genes, Ofd1 and Bbs4 , leads to a reduction in glucose-stimulated first phase insulin secretion in murine pancreatic islets and in a β-cell line. At the same time, there was no significant change in KCl-stimulated insulin secretion, suggesting that the observed phenotype is glucose-specific rather than a global exocytotic defect. In vivo , we found a reduced acute insulin response when we challenged Bbs4 −/− mice with glucose. This effect is likely cilia specific. Third, basal body/ciliary defects should compromise at least one of the known signalling networks involved in (pre-) diabetic phenotypes. Altered IR signalling has been observed in human islets from T2DM patients [53] . Loss of first phase insulin secretion has also been reported for the βIRKO mouse, a T2DM susceptibility model. In localization studies on a β-cell line and primary human β-cells, we showed that IR is recruited to the primary cilium of insulin-stimulated β-cells and that this recruitment is necessary for proper insulin signal transduction. In a β-cell line and in whole islets, disruption of Ofd1 and Bbs4 leads to decreased activation of two major nodes of the insulin signalling network, the p85/p55 regulatory subunits of PI3-kinase and the serine/threonine kinase Akt. A reduction of SNARE proteins has been reported in PI3K- signalling-deficient mice [42] and preassembled t-SNARE complexes have been implicated in first phase insulin secretion [44] . We found a reduction in SNARE components Snap25 and Syntaxin1A, both targets of PI3K/FoxO1 transcriptional regulation. Reduced levels of one or more SNARE component could shift the steady-state equilibrium in the β-cell and specifically reduce the number of preassembled SNARE complexes. Re-introduction of STX1A partially rescues insulin secretion and supports a role for p85/p55-dependent transcriptional regulation in first phase insulin release as well as ciliary signalling. Critical signalling nodes such as Akt or PI3K are highly regulated (positively and negatively) and represent junctions for potential crosstalk with other signalling networks [38] . Both Akt and PI3K are components of a variety of signalling cascades and we cannot exclude that basal body/ciliary disruption will affect other pathways that converge at the nodes of PI3K and Akt kinases thus accounting for some of the observed differences in phosphorylation levels. Fourth, models of T2DM should show evidence of ciliary defects. In GK rats, we observed a roughly threefold reduction in primary cilia on β-cells. In addition, we also found several ciliary/basal body genes to be misexpressed in GK islets. Moreover, we confirmed a reduction of Stx1a protein in GK islets. Similarly, several ciliary/basal body genes have been shown to be misregulated in pancreatic islets of another diabetes model, ob/ob mice [54] , further supporting a role for cilia in T2DM. In summary, our data strongly suggest a link between ciliary dysfunction and T2DM susceptibility. To our knowledge, this is the first study to address the role of primary cilia in glucose handling, insulin signalling and T2DM susceptibility. Moreover, it is also one of the first to investigate the role of cilia in pancreatic tissue homeostasis. Hence, our findings further the understanding of the disease mechanism underlying T2DM and present a novel approach for therapeutic intervention. For all experiments with human material, informed consent was obtained; they were carried out in concordance with the Swedish ethical regulations. Experiments involving human islets were approved by the Regional Ethics Review Committee Stockholm, Department III. All experiments on animals were carried out in concordance with the ethical regulations on laboratory animals and ethical approvals of the Animal Ethics Committee Stockholm-North. Statistical tests Unless stated otherwise, we used Student’s t -tests to assess statistical significance. For comparison of more than two groups, we ran outlier analyses (Grubbs, where applicable) and used one-way ANOVA tests. Design and synthesis of shRNA adenoviral constructs Two target sequences per gene of interest ( Mus musculus ) were chosen (one in the open reading frame, one in the 3′UTR): For Ofd1 5′- GCTAGAATCTTTAGAGACA -3′ (shOfd1_A)/5′- GCACTTTGTTACTGAGATT -3′ (shOfd1_B), and for Bbs4 5′- GGATAAAGCCATCGAGATC -3′ (shBbs4_A) and 5′- GTTGAGACCTAGATGGAAT -3′ (shBbs4_B). The corresponding oligonucleotides were ligated into the entry vector for the ViraPower Adenoviral expression system (pENTR, Life Technologies) according to the manufacturer’s instructions. The efficacy was assessed according to relative level of message by quantitative reverse transcription–PCR. The most efficient shRNA was then shuttled into the adenoviral expression vector and viral stock generated according to the manufacturer’s specifications (Life Technologies). For reasons of clarity, we refer to more effective shRNA construct shOfd1_A as shOfd1 and shBbs4_B as shBbs4 in the text. Blood glucose and serum insulin level in Bbs4 mice To produce homozygous Bbs4 knockout (−/−) and littermate control (+/+), heterozygous mice with a mixed genetic background of C57BL/6J and 129/SvEv were crossed. For fasting glucose and insulin test, animals were fasted for 12 h. Glucose was measured with Accu-Chek compact plus monitoring system (Roche Diagnostics). Serum insulin was measured by mouse insulin ELISA kit (Crystal Chem Inc.). Quantitative reverse transcription–PCR MIN6m9 cells were seeded (800,000 cells per 6 cm dish) and cultured overnight. Next day, they were transduced with adenoviral constructs targeting the genes of interest or expressing scrambled RNA, respectively, in duplicates. After 24 h, cells were washed and seeded into six-well dishes (225,000 per well) and the culture medium changed to OptiMEM (Life Technologies) 48 h post transduction. Another 48 h later, cells were treated with 5 mU ml −1 insulin in OptiMEM or fresh OptiMEM for 3 min, respectively; after stimulation, cells were washed with OptiMEM (twice) and cultured for 1 h before harvesting. Total RNA was isolated using the RNeasy kit from Qiagen according to the manufacturer’s specifications. mRNA was transcribed into cDNA using the SuperScript III First Strand kit from Invitrogen. Ins , βGCK , Kif3a , Ofd1 and Rsd3 messages were quantified using the SYBR Green kit from Life Technologies on an ABI Prism 7900 from BD Biosciences (for primer sequences, please refer to Supplementary Table 1 ). Ins and βGCK messages were normalized to those of unstimulated cells. Pancreatic islets from GK and Wistar rats were cultured for 24 h after isolation. The tissue was homogenized with a Dounce homogenizer and RNA isolated using the RNeasy Micro kit (Qiagen). Ciliary and basal body gene expression levels were monitored using TaqMan assays for Ift88 (Rn01489251_m1), Bbs4 (Rn01766633_m1) and Pcm1 (Rn01488002_m1) and normalized to 18S (100 fold dilution of the template) with TaqMan Fast Advanced Master Mix (all BD Biosciences/Applied Biosystems) on an ABI Prism 7900HT system. ELISA Quantification of pSer473 Akt to pan-Akt ratios was carried out on stimulated cells or islets using an ELISA kit (ab126433, Abcam) according to the manufacturer’s instructions. Pancreatic sections from GK and Wistar rats Pancreata were swiftly removed from euthanized animals, washed in PBS and fixed in 4% paraformaldehyde in PBS overnight. Pancreata were then washed with PBS (x2) and transferred to 10% sucrose in PBS. After 24 h, the tissue was moved to 20% sucrose and to 30% sucrose another 5 h later. It was washed briefly with PBS and then frozen in O.C.T. freezing medium (Fisher Scientific) at −80 °C and subsequently sectioned into 20-μm thick sections. Image analysis The rat pancreatic islet image volume was analysed using MATLAB (Mathworks). The image was globally thresholded using Otsu’s method [55] , and the resulting binary volume is then morphologically opened using a 3 × 3 × 3 structuring element to reduce noise. The distance to the background for each object voxel in the opened image is calculated using a distance transform with the Euclidean metric. Each object is individually labelled, and objects with a maximal distance smaller, or equal, to 2.0 voxels are further identified. An output image volume, with the same size as the input image, is created having a black background. Small objects selected for manual discrimination are visualized in the output image with a light grey intensity, and the remaining objects are given a dark grey intensity. The original image volume is then manually investigated with the output image volume as an overlay, thus indicating small interesting structures. The image volumes and overlays were analysed in Volocity (Improvision/Perkin Elmer). The ROI was selected based on insulin staining and the volume of insulin-positive structures calculated. Acetylated-tubulin-positive structures in the ROI that are touching the borders of the ROI were excluded from further analysis. In addition, structures larger than 50 μm 3 as well as those more than 15 μm in length were automatically excluded. The remaining structures were individually investigated. Cilia were counted and their skeletal length recorded. In the final data analysis, we excluded insulin-positive volumes of less than 100,000 μm 3 to avoid sections in the periphery of the islet. Cell and tissue culture MIN6m9 cells were cultured in DMEM (GIBCO, Life Technologies) supplemented with 10% fetal bovine serum (FBSGIBCO), 1 g l −1 D -glucose (Sigma Aldrich) and 5 μl l −1 β-Mercaptoethanol (Sigma Aldrich). Islets were isolated from age-matched 4- to 5-month-old male C57B6 mice (Charles River) according to a previously published protocol [56] . Isolated islets were cultured in RPMI-1640 (GIBCO) supplemented with 10% FBS and Penicillin/Streptomycin. Nocodazole (CAS# 31430-18-9) and Colchicine (CAS# 64-86-8) were purchased from Biotrend Chemikalien GmbH. Human islets were dispersed with Accutase (GIBCO) and cultured in CMRL 1066 medium (GIBCO) supplemented with 25 mM HEPES, 50 U penicillin/streptomycin, 2 mM L -glutamine, 5 mM nicotinamide and 10% FBS. Cells were treated with 100 nM nocodazole for 6 h or 2 μM colchicine for 4 h, respectively. XF Extracellular flux analysis Metabolic flux analysis was performed using Seahorse XF24 Extracellular Flux Analyser (Seahorse Biosciences). Two days after transduction, 30,000 cells per well were seeded. The next day the growing medium was replaced with XF medium, containing 2 mM GlutaMax (GIBCO) and 2% FBS. Cells were incubated at 37 °C without CO 2 1 h before the experiment. We measured the rates before (baseline) and after addition of glucose (11 mM final concentration). The running template included: 2 min mix, 1 min delay and 4 min measure. Data are presented using baseline normalization. Glucose uptake Two days after transduction, 200,000 cells per well were seeded using growing medium and starved overnight in OptiMEM. The next day the medium was replaced with OptiMEM containing 11 mM glucose and 5 μl ml −1 of deoxy- D -glucose, 2-[1,2-3H(N)] (Perkin-Elmer) for 1 h. Cells were then washed three times with saline solution and 400 μl of lysis buffer (1%SDS in 0.1 M NaOH) were added. The lysate was shaken for 1 h and recollected. The radioactive count was performed using a Wallac 1409 liquid scintillation counter (Perkin-Elmer). Glucose levels were normalized to protein (Lowry). IR localization After dispersion, human islet cells were cultured in CMRL medium for 24 h and subsequently starved in OptiMEM medium for 48 h. Cells were stimulated with 5 mU ml −1 human insulin at 37 °C for 3 min and then pre-extracted in 60 mM PIPES, 25 mM HEPES, 10 mM EGTA and 4 mM MgSO 4 with 0.5% Triton-X for 30 s before fixation with 3% paraformaldehyde in PBS at room temperature (RT) for 30 min. After post-fixation in ice-cold methanol at −20 °C for 10 min, cells were blocked in 1% blocking reagent (Life Technologies) in PBS with 0.1% Triton-X at RT. MIN6m9 cells were seeded onto coverslips (75,000 per coverslip) and cultured overnight. They were transfected with pRcCMVi IR A-Flag, pRcCMVi IR B-Flag, pRcCMVi IR A KD-Flag [47] , [48] or pRcCMVi IR A V938D or pRcCMVi IR B V950D, respectively, using Lipofectamine (Life Technologies) according to the maunfacturer’s specifications and cultured in OptiMEM. After 48 h, cells were treated with 5 mU ml −1 human insulin in OptiMEM or fresh OptiMEM for 3 min at 37 °C. Subsequently, cells were washed with PBS and fixed (see below). Co-distribution was assessed as follows: cilia were considered positively correlated with IR when the outline of the cilium (acetylated α-tubulin, red) could be appreciated in the IR (green) channel. Immunofluorescent staining Cells or islets were fixed in ice-cold methanol (−20 °C,10 min) or 3% paraformaldehyde solution (RT, 30 min). They were permeabilized in 0.1% Triton-X in PBS, blocked with 5.5% FBS or 10% goat serum in PBS, respectively, and incubated with primary antibodies: anti-detyrosinated α-Tubulin (rabbit, 1:500, Abcam, ab48389), anti-α-Tubulin (mouse, 1:1,000, Sigma-Aldrich, T6199), anti-γ-tubulin (mouse, 1:1,000, Sigma-Aldrich, T6557), anti-acetylated tubulin (mouse, 1:1,000, Sigma-Aldrich, T6793), anti-insulin (chicken, 1:1,000, Abcam (out of stock) or guinea-pig, 1:250, Abcam, ab7842)), anti-Flag (rabbit polyclonal, 1:1,000, Abcam, ab21536), anti-IR (rabbit polyclonal, 1:400, Biodesign) or anti-IR-B (rabbit polyclonal, 1:400, Biodesign), anti-Arl13b (rabbit polyclonal, 1:100, Acris Antibodies) or anti-GFP (chicken, 1:2,000, Abcam, ab13970) at RT for 1 h or at 4 °C overnight. After washing with PBS, cells were incubated with secondary antibodies (goat anti-rabbit IgG H+L Alexa Fluor 633, goat anti-mouse IgG H+L Alexa Fluor 488 or 633, goat anti-chicken IgG H+L 488; all Life Technologies) at RT for 1 h. For the detection of endogenous insulin-receptors using anti-IR and anti-IR-B, the TSA-amplification kit #12 (anti-rabbit, Alexa488; Life Technologies, t-20922) was utilized according to the manufacturer’s instructions. Cells were mounted in ProLong Antifade Gold (Life Technologies) and imaged on Leica DM EFSA and DM IRBE Confocal Microscopes at × 20, × 63 or × 100 magnification. Confocal laser scanning microscopy of endogenous IR in MIN6m9 cells was performed on a LEICA SP2 using the following settings: objective lens × 100, 1.4 numerical aperture, double-dichroic mirror 488/546, between lines sequential scan, detection of Alexa 488 (label for IRs) excitation 488 nm, emission 500–520 nm; detection of Alexa 546 (label for cilia) excitation 546 nm, emission 560–620 nm. Shown are single confocal images unless indicated otherwise. Tissue sections were treated with ice-cold methanol at −20 °C for 30 min, washed in PBS twice and then permeabilized in 0.05% Saponin (Sigma Aldrich) in PBS at RT for 1 h. Sections were blocked with 10% goat serum in PBS with 0.1% Triton-X at RT for 1 h or at 4 °C overnight and incubated with a mixture of anti-acetylated tubulin (mouse, 1:500, Sigma-Aldrich, T6793) and anti-insulin (guinea-pig, 1:250, Abcam, ab7842) at 4 °C overnight. After washing with PBS (three times), the tissue was incubated with a mixture of goat anti-guinea pig IgG (H+L) Alexa Fluor 546 (1:1,000, Life Technologies) and goat anti-mouse IgG2B Alexa Fluor 647 (1:1,000, Life Technologies) in PBS with 0.1% Triton-X at RT for 4 h and then mounted with Prolong Antifade Gold (Life Technologies) and imaged on a Leica DM EFSA confocal microscope with sequential scanning of laser wavelengths 546 nm and 633 nm at × 100 magnification (1.4 numerical aperture). Glucose tolerance Before the measurements, animals were fasted for 12 h. Because of the anxiety phenotype of Bbs4 −/− animals [15] , we sedated both wild-type and knockout animals with very low doses of Hypnorm (VetaPharma Ltd.)/Dormicum (F.Hofmann-LaRoche Ltd; 1/16 of the dose to induce surgical anaesthesia; 5 μg ml −1 fentanyl, 156 μg ml −1 fluanison, 250 μg ml −1 midazolam in water; 100 μl per 10 g bodyweight) 60–90 min before the procedure [57] . Animals were calm but responsive and moving in their cages during the procedure. We injected 2 g kg −1 glucose (20% glucose solution) intraperitoneally. Blood glucose values were measured using an Accu-Check system (Roche Diagnostics). During the first 20 min, we removed blood samples at predefined time points for serum insulin measurements (ArcDia). Rescue experiments MIN6m9 cells were plated (150,000 cells per 3.5 cm dish) and incubated in growth medium (37 °C, overnight). The following day, cells were treated with adenoviral shRNA constructs and, 24 h post treatment, transfected with 800, 1,600 or 2,400 ng of pCMV mycBBS4 (human ORF) or pCRII Stx1a, respectively. We used empty vector (pCMVmyc) to keep the plasmid DNA levels constant. Lipofectamine 2000 was used as a transfection reagent according to the manufacturer’s specifications (Life Technologies). The cells were washed with PBS and incubated in growth medium the day following transfection. 48 h post transfection, we incubated the cells in 0.5 mM KRBH buffer (115 mM NaCl, 4.7 mM KCl, 1.2 mM K 2 HPO 4 , 1.2 mM MgSO 4 , 20 mM NaHCO 3 , 16 mM HEPES, 2.56 mM CaCl 2 , 0.1 g l −1 BSA, pH 7.4) at 37 °C for 1 h before the assay. Western blots 15 min post stimulation (5 mU ml −1 insulin) islets were lysed in modified RIPA buffer (150 mM NaCl, 50 mM Tris-HCl pH 7.4, 1% NP-40, 0.1% sodium deoxycholate, 1 mM EDTA) supplemented with protease and phosphatase inhibitors (Mini Complete/PhosphoStop, Roche Diagnostics). Protein content was measured using the BCA method (Pierce, Thermo Fisher Scientific). Protein extracts were separated on NuPage Bis Tris 4–12% minigels (Life Technologies) and transferred to PVDF membranes. Blots were probed with γ-tubulin antibody (1:1,000, s.a.), Pcm1 antibody (1:200, ab72443, Abcam), Phospho Akt (pSer473, Cell Signaling, #4060, 1:1,000), pan-Akt (Cell Signaling #4685, 1:1,000), phospho p85/p55 (pTyr458/199) (Cell Signaling #4228, 1:1,000) and secondary anti-mouse/-rabbit IgG (H+L)-HRP conjugates (1:5,000, GE Healthcare). Quantification was carried out on scanned films using ImageJ and normalization to loading control (γ-tubulin). Experiments were carried out in triplicate unless noted otherwise. How to cite this article: Gerdes, J. M. et al . Ciliary dysfunction impairs beta-cell insulin secretion and promotes development of type 2 diabetes in rodents. Nat. Commun. 5:5308 doi: 10.1038/ncomms6308 (2014).